WDM-compatible mode-division multiplexing on a silicon chip Significant effort in optical-fibre research has been put in recent years into realizing mode-division multiplexing (MDM) in conjunction with wavelength-division multiplexing (WDM) to enable further scaling of the communication bandwidth per fibre. In contrast, almost all integrated photonics operate exclusively in the single-mode regime. MDM is rarely considered for integrated photonics because of the difficulty in coupling selectively to high-order modes, which usually results in high inter-modal crosstalk. Here we show the first microring-based demonstration of on-chip WDM-compatible mode-division multiplexing with low modal crosstalk and loss. Our approach can potentially increase the aggregate data rate by many times for on-chip ultrahigh bandwidth communications. Current-integrated photonics operate almost exclusively in the single-mode regime and utilize wavelength-division multiplexing (WDM) [1] , [2] , which supports limited scalability in bandwidth density. In contrast, fibre communications are increasingly targeting multimode operation in conjunction with WDM to further scale the communication bandwidth transmitted per fibre [3] . Multimode communications in fibres have been demonstrated with space-division multiplexing in multi-core fibres [4] , [5] , [6] , [7] , [8] or mode-division multiplexing (MDM) in few-mode fibres [9] , [10] , [11] , [12] , [13] , [14] , [15] , [16] , [17] and have exploited each spatial mode as an independent channel. It is similarly of interest to attempt to incorporate the spatial-mode-parallelism degree of freedom into complex photonic-integrated circuits to introduce additional functionality and provide potential performance gains. In particular, one application of interest for photonic-integrated circuits is on-chip and off-chip high-bandwidth-density interconnects. Here we present a platform enabling MDM in conjunction with WDM for such on-chip photonic networks. This platform could increase the bandwidth density of on-chip interconnects without increasing the number of waveguides, waveguide crossings (which can dominate the loss in complex interconnects [18] , [19] ) and chip area, as well as add an additional design degree of freedom in future photonic-integrated circuits and networks. Some of the key challenges of realizing on-chip MDM-enabled interconnects lie in creating mode (de)multiplexers with low modal crosstalk and loss, which also support WDM (a key feature of many integrated-optics interconnect designs). Previous implementations of on-chip mode multiplexers based on Mach–Zehnder interferometers [20] , [21] , Multimode Interference couplers [22] , [23] , [24] , asymmetric directional couplers [25] , [26] , [27] and y-junctions [28] , [29] , [30] typically had large footprints, complex and strict design limitations or only supported a limited number of optical modes. A compact and reconfigurable mode (de)multiplexer that can be straight-forwardly scaled to support numerous modes is essential for realizing MDM–WDM in integrated photonics. In the following sections, we detail the first microring-based demonstration of an on-chip WDM-compatible mode-division multiplexing (and demultiplexing) scheme. The system performance of this scheme with all of its associated stages (multiplexing, transmission and demultiplexing) is characterized with multiple co-propagating 10 Gb s −1 high-speed communication signals reaching up to 60 Gb s −1 of aggregate bandwidth. Selective mode coupling by phase matching We demonstrate on-chip MDM–WDM by engineering the propagation constants of high-confinement photonic structures in order to enable selective coupling to different spatial modes at different wavelengths. The silicon photonic platform is attractive for implementing this approach as the propagation constants of the different spatial modes can be engineered to differ significantly—thanks to the high core-cladding (Si/SiO 2 ) index contrast. We choose a waveguide height for which the confinement is high, and therefore widely different propagation constants can be achieved by varying the waveguide width. 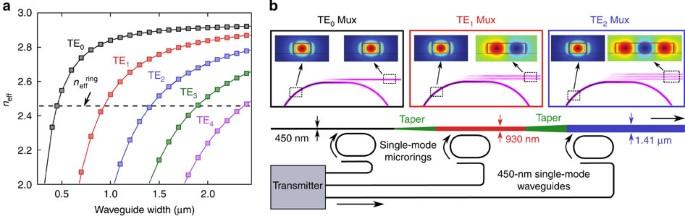Figure 1: Phase-matching condition for 250-nm-tall silicon waveguides. (a) Simulated effective index of the optical modes in waveguide of different widths atλ=1,550 nm. (b) Selective coupling of the single-mode microrings to a specific spatial mode in the multimode waveguide, with each section of the multimode waveguide linked by adiabatic tapered waveguides. The insets show the selective coupling of each multiplexer (TE0, TE1and TE2). Figure 1a shows that for a given 250-nm-tall silicon waveguide a large range of effective indices from 2.0 to 2.9 can be achieved corresponding to the propagation constants of the TE 0 (transverse electric) through TE 4 spatial modes at λ =1,550 nm. On the basis of propagation constant matching, an optical mode in a single-mode waveguide can be evanescently coupled to a specific spatial mode in an adjacent multimode waveguide, in which the coupling strength to the mode depends on the width of the multimode waveguide. Figure 1: Phase-matching condition for 250-nm-tall silicon waveguides. ( a ) Simulated effective index of the optical modes in waveguide of different widths at λ =1,550 nm. ( b ) Selective coupling of the single-mode microrings to a specific spatial mode in the multimode waveguide, with each section of the multimode waveguide linked by adiabatic tapered waveguides. The insets show the selective coupling of each multiplexer (TE 0 , TE 1 and TE 2 ). Full size image In order to realize a compact and tunable MDM device, we employ single-mode microring resonators to selectively couple to the different spatial modes in a multimode waveguide. To simultaneously support multiple WDM channels in the MDM scheme, we design the free-spectral range of the microrings to match the wavelength channel spacing. The mode multiplexer and demultiplexer, which are designed to operate in the quasi-TE mode, comprise of three identical microrings coupled to a multimode waveguide (see Fig. 1b ). Each microring, formed from a 450-nm-wide waveguide, is designed to support only the fundamental TE mode with an effective index of 2.46. The multimode transport waveguide comprises several sections with tapering widths ranging from 450 nm to 1.41 μm. When the multimode waveguide width corresponds to 450 nm, 930 nm or 1.41 μm, the effective indices of TE 0 , TE 1 or TE 2 modes, respectively, match the effective index of the TE 0 mode of the microrings ( n eff =2.46) and therefore couple efficiently to the microrings. The three insets in Fig. 1b show such coupling of the TE 0 mode of the microring to the TE 0 , TE 1 or TE 2 modes in the multimode waveguide. In order to achieve good device performance, the coupling through the microrings has to minimize the insertion loss for the desired mode as well as minimize the power coupled to the other modes. This can be achieved by optimizing the coupling gap and coupler length between the microrings and the waveguides. For example, with a 200-nm gap (see Fig. 2a ), the power coupled from the microring to the modes of a 1.41-μm waveguide can be computed based on the coupled-mode analysis (see Methods) as depicted in Fig. 2b . With the microring-based design, a short coupling length is feasible as only a relatively low coupling strength is required to transfer all the power from the single-mode input waveguide to the TE 2 mode in the multimode drop waveguide via the microring (typically termed critical coupling) [31] . The coupling to the undesired modes (TE 1 and TE 0 ) is much weaker because of the phase mismatch of these modes, and thus a 6-μm-long coupling length can achieve optimal loss and crosstalk performance (see Fig. 2c ). 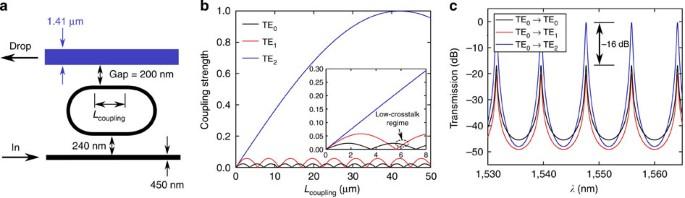Figure 2: Coupling strength of the three spatial TE modes of a 1.41-μm-wide waveguide to the TE0mode of a 450-nm-wide microring waveguide. (a) Schematic of an add-drop microring with asymmetric input and drop waveguides. (b) Calculated coupling strength of the coupling region between the microring and the multimode waveguides. The inset shows the zoom-in coupling strength for coupling length <8 μm. A short coupling length (low coupling strength) is sufficient to achieve critical coupling between the single-mode input waveguide and the multimode drop waveguide via the microring. (c) Simulated transmission and crosstalk levels at the drop port with an optimized coupling length of 6 μm. Figure 2: Coupling strength of the three spatial TE modes of a 1.41-μm-wide waveguide to the TE 0 mode of a 450-nm-wide microring waveguide. ( a ) Schematic of an add-drop microring with asymmetric input and drop waveguides. ( b ) Calculated coupling strength of the coupling region between the microring and the multimode waveguides. The inset shows the zoom-in coupling strength for coupling length <8 μm. A short coupling length (low coupling strength) is sufficient to achieve critical coupling between the single-mode input waveguide and the multimode drop waveguide via the microring. ( c ) Simulated transmission and crosstalk levels at the drop port with an optimized coupling length of 6 μm. Full size image We design the microring resonance linewidth to be at least 15-GHz in order to enable 10-Gb s −1 data transmission with negligible signal degradation. We also include an integrated heater on top of each microring to tune the microring resonances to align to the WDM channels and thereby optimize the performance of the device [32] . This design can be easily modified to handle additional phase-matched modes by widening the multimode waveguide ( Fig. 1a ). In this particular design scheme, the multimode transport waveguide width is varied, requiring the lowest order mode to be added first and dropped last. However, one could in principle keep the multimode waveguide width constant and instead vary the microring waveguide width, enabling the addition and dropping of arbitrary modes without disturbing neighbouring modes. Another direct extension of this design is the inclusion of additional sets of identical microrings coupled to each multimode waveguide section to enable wavelength-channel grooming directly on each spatial mode. Optical performance of the fabricated device The fabrication details for this MDM device ( Fig. 3a ) are documented in the Methods section. We image the optical modes at the output of the multimode waveguide to verify the excitation of the different spatial modes (see Methods for the imaging experimental details). We observe well-defined TE 0 , TE 1 and TE 2 modes as predicted by simulation ( Fig. 3b ). From the spectral transmission scans for each combination of input and output ports, we can quantify the amount of crosstalk resulting from the spatial mode multiplexing and demultiplexing. 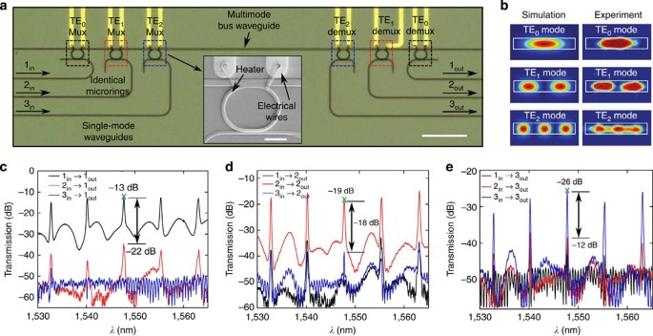Figure 3: Optical performance of the fabricated device. (a) Microscope image of the fabricated device (100 μm scale). Inset: scanning electron microscope (SEM) image showing the heater to tune each individual microring resonator (10 μm scale). (b) Simulated and experimental images of the optical modes at the cross-section of the multimode waveguide. (c–e) Optical transmission and crosstalk at the three output ports for signal injection on each of the three input ports. Figure 3c shows the transmission spectrum at output port 1 (see port definitions in Fig. 3a ) from each input. The measured insertion loss of this port at λ =1,547 nm is 13 dB and the optical crosstalk (defined as the ratio of desired signal power to the sum of the interfering channels’ power) is −22 dB. The insertion loss of port 2 at λ =1,547 nm is 19 dB and the optical crosstalk is −18 dB ( Fig. 3d ). The insertion loss of port 3 at λ =1,547 nm is 26 dB and crosstalk is −12 dB ( Fig. 3e ). The main contribution to the insertion loss is the aggregate 10-dB fibre-to-chip coupling loss. The rest of the insertion loss is attributed to the waveguide propagation loss and microring intrinsic loss. The higher insertion loss in port 3 compared with the other two ports is because of a suboptimal microring coupling gap. By ensuring critical coupling between the waveguides and microrings, achievable on-chip losses of this device are expected to total around 1.5 dB. Figure 3: Optical performance of the fabricated device. ( a ) Microscope image of the fabricated device (100 μm scale). Inset: scanning electron microscope (SEM) image showing the heater to tune each individual microring resonator (10 μm scale). ( b ) Simulated and experimental images of the optical modes at the cross-section of the multimode waveguide. ( c – e ) Optical transmission and crosstalk at the three output ports for signal injection on each of the three input ports. Full size image As detailed in the previous section, the crosstalk can be minimized by optimizing the coupling length between the microring and the multimode waveguide to reduce coupling of the undesired modes (see Fig. 2b ). We expect the crosstalk at the output port 3 of the current device to be less than −16 dB for an optimized coupling length of 6 μm (the fabricated coupler was only 5 μm long) (see Fig. 2c ). The crosstalk can be further reduced by introducing weaker coupling at the microring–multimode waveguide coupling region (by having a larger coupling gap of 280 nm) to lower the maximum coupling of the undesired modes. This in turn results in a longer coupling length ( L coupling ≈11 μm) to maintain the critical coupling condition and from our calculations should enable devices with less than −30 dB of crosstalk. High-speed MDM link with three spatial modes We simultaneously launch a single 10-Gb/s data channel into all the three input ports of the mode multiplexer and measure a small power penalty (<1.9 dB measured at a BER of 10 −9 ) on each output port of the mode demultiplexer. The experimental setup for performance evaluation is illustrated in Fig. 4a . In order to measure these power penalties, the laser channel at 1,563 nm is modulated with PRBS 2 31 −1 on-off-keyed data by an amplitude modulator and then further phase-imprinted with a swept-frequency sinusoid in order to enable bit-error-rate (BER) measurements on channels that experience coherent crosstalk (further information is provided in the Methods section). The data signal is then amplified, split evenly between the three input ports of the on-chip mode multiplexer and simultaneously injected in quasi-TE polarization to the multiplexer ports. The varying fibre spans leading to the device ensure that the data are decorrelated between the ports (see Methods). The demultiplexed signals are recovered one at a time for inspection on a DCA and BER evaluation. Error-free transmission (BER <10 −12 ) and open eye diagrams ( Fig. 4b,c ) are observed for all the signals at the three output ports. To account for fabrication imperfections, we improve the performance of port 3 at the expense of increased crosstalk and spectral filtering penalties on port 2 by wavelength detuning the TE 1 multiplexer microring. This enables device operation with an overall balanced power penalty of 1.9 dB on ports 2 and 3 and 0.5 dB on port 1. In order to verify that the intrachannel crosstalk is indeed the main mechanism of signal degradation [33] , we also inspect the channel performance with only one input port injected at a time. We observe that the single-input transmission results in 0.1 dB penalties on ports 1 and 2 and 0.8 dB on port 3 (with the higher penalty on port 3 resulting from the higher insertion loss through this port, which leads to a larger OSNR degradation at the post-chip EDFA). Therefore, we conclude that crosstalk is the main contributing factor to signal degradation in this device. The penalties are measured relative to a back-to-back reference case, which is defined and measured by replacing the chip with a tunable attenuator set to replicate the fibre-to-fibre loss of the lowest insertion-loss port. 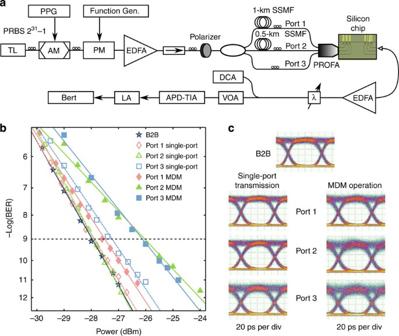Figure 4: 3-Mode × 10 Gb s−1multiplexing link. (a) Experimental setup for performance evaluation including Pulsed Pattern Generator (PPG), Tunable Laser (TL), Amplitude Modulator (AM), Phase Modulator (PM), Erbium-Doped Fibre Amplifier (EDFA), Isolator (→), Standard Single-Mode Fibre (SSMF), Tunable Filter (λ), Digital-Communications Analyzer (DCA), Variable Optical Attenuator (VOA), Avalanche-Photodiode (APD-TIA), Limiting Amplifier (LA) and Bit-Error-Rate Tester (BERT). (b) BER measurements for back-to-back (B2B) test case, single port transmission and MDM operation for all three ports. (c) Corresponding eye diagrams for the inspected signals. Figure 4: 3-Mode × 10 Gb s −1 multiplexing link. ( a ) Experimental setup for performance evaluation including Pulsed Pattern Generator (PPG), Tunable Laser (TL), Amplitude Modulator (AM), Phase Modulator (PM), Erbium-Doped Fibre Amplifier (EDFA), Isolator (→), Standard Single-Mode Fibre (SSMF), Tunable Filter ( λ ), Digital-Communications Analyzer (DCA), Variable Optical Attenuator (VOA), Avalanche-Photodiode (APD-TIA), Limiting Amplifier (LA) and Bit-Error-Rate Tester (BERT). ( b ) BER measurements for back-to-back (B2B) test case, single port transmission and MDM operation for all three ports. ( c ) Corresponding eye diagrams for the inspected signals. Full size image MDM–WDM link with two spatial modes and three WDM channels We measure a low (<1.4 dB) power penalty for joint MDM–WDM operation by launching three different 10-Gb/s wavelength channels spanning the full C-band into two input ports of the multiplexer (ports 1 and 2). A modified setup (depicted in Fig. 5a ) is used to correctly decorrelate the wavelength channels (see Methods), and polarizers are included in the experiment to ensure that all the wavelength channels are launched on chip at the quasi-TE polarization with equal power. We set the wavelength channels to span the full C-band (limited by the EDFA gain band) and the microrings are tuned on-resonance to maximize power transmission at 1,547 nm. The power penalties for both ports vary between 0.6 and 1.4 dB for all the three wavelength channels ( Fig. 5b ) with performance variation attributed to slightly varying levels of crosstalk for the different wavelength channels. Error-free transmission (BER <10 −12 ) and open eye diagrams ( Fig. 5c ) are observed for all the three channels at the two output ports. These results show that only a minimal penalty is added by extending the device operation to support WDM concurrently with the MDM. 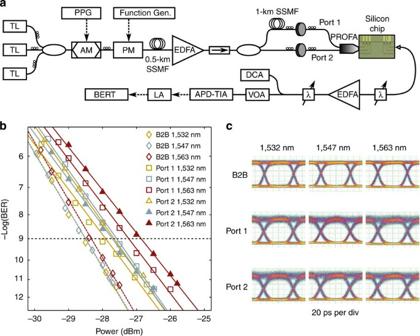Figure 5: 2-Mode × 3-wavelength × 10 Gb s−1MDM–WDM link. (a) Experimental setup for demonstrating combined MDM and WDM operation. (b) BER measurements for B2B test cases and full MDM–WDM operation for both ports. (c) Corresponding eye diagrams for the inspected signals. Figure 5: 2-Mode × 3-wavelength × 10 Gb s −1 MDM–WDM link. ( a ) Experimental setup for demonstrating combined MDM and WDM operation. ( b ) BER measurements for B2B test cases and full MDM–WDM operation for both ports. ( c ) Corresponding eye diagrams for the inspected signals. Full size image In conclusion, we have shown a platform that enables on-chip MDM–WDM optical interconnection for ultrahigh bandwidth communications. Our simulation in Fig. 1a showed that when the multimode waveguide width tapers up to 2.37 μm, five spatial modes can be supported by this platform. In principle using a wider waveguide one could support an even larger number of modes. Each microring resonator in practice is able to support 87 WDM channels over the entire C-band (1,530–1,565 nm) by increasing the microring size such that the channel spacing is 50 GHz. Therefore, the on-chip MDM–WDM platform with the above-mentioned dimension design can potentially support an aggregate data rate up to 4.35 Tb s −1 with five spatial modes and 87 WDM channels. Device design and fabrication We fabricate the reconfigurable MDM–WDM silicon microring resonators on a 250 nm SOI wafer with 3 μm of buried oxide using standard CMOS fabrication processes. We patterned the waveguides using e-beam lithography with the dimensions as followed: the input/output ports and the microring are 450 nm wide; the TE 0 , TE 1 and TE 2 (de)multiplexers multimode transport waveguide are 450 nm, 930 nm and 1.41 μm wide, respectively, and each (de)multiplexer is linked by an adiabatic taper of 80 μm long. All the microrings have a radius of 10 μm and a coupling length of 5 μm. The separation gap between the microrings and all the input waveguides is 240 nm, while the separation gaps between the microrings and TE 0 , TE 1 and TE 2 (de)multiplexer multimode waveguide are 240 nm, 200 nm and 200 nm, respectively. The silicon waveguides are then etched, followed by the e-beam resist being stripped and the etched structures are clad with a 1-μm-thick silicon oxide layer using plasma-enhanced chemical vapour deposition to confine the optical mode. NiCr (300 nm) is subsequently evaporated on the microring resonators above the cladding to create the 1-μm-wide heaters. Finally, 500 nm of gold (Au) are evaporated to define the electrical wires and contact pads using a lift-off process. The final fabricated device is illustrated in Fig. 3a . The footprint of this device is 0.11 mm 2 excluding the electrical wires. Imaging of the spatial modes in the multimode waveguide We fabricate a test device that only has the mode multiplexer section (TE 0 , TE 1 and TE 2 ) and is terminated with the 1.41-μm wide multimode waveguide. We couple a 1,547-nm laser (on-resonance of each microring) into one of the input ports at one time. The output spatial modes of the multimode waveguide are then magnified with a × 40 aspheric lens and imaged on an infrared camera as shown in Fig. 3b . Coupled-mode analysis for asymmetric coupled waveguides Coupled-mode theory for two weakly coupled optical modes relates the complex amplitudes of the modes a 1 and a 2 through a set of differential equations [34] : the solutions to this equation set, assuming the waves a 1 (0) and a 2 (0) are launched at z =0, are given by: where If the initial waves a 1 (0)=1 and a 2 (0)=0 are assumed, then the coupling from a 1 to a 2 is given by . Phase dithering Intrachannel crosstalk [33] results in coherent interference of the laser with itself. In a test setup not employing any phase decoherence mechanisms, this results in a slow change of the output signal power as the phases leading to the device under test change as a result of thermal fluctuations in the fibres. If this remains untreated, these power fluctuations (on the temporal order of multiple seconds) prevent accurate BER measurements over short time spans. In order to enable finite-time BER measurements, two mechanisms are employed simultaneously to average out the slow phase fluctuations: (1) the arms leading to the multiplexer input ports are decorrelated by at least 0.5 km Standard Single-Mode Fibre. This is close to the 1-km coherence length of the 200-kHz linewidth lasers we used in the experiments, therefore ensuring some phase decoherence of the signals. (2) In order to guarantee full-phase orthogonality regardless of the intrinsic laser linewidth, we incorporate phase modulation of a repeating linearly chirped signal consisting of a frequency sweep from 20 to 10 MHz over a 5-ms period. With a 0.5-km path difference (roughly 2.5-s relative delay), the phase difference between adjacent ports oscillates over 2 π at 5 kHz, guaranteeing averaging of the phase difference in power measurements averaged over 100 ms. Multiport edge coupling Employing a method similar to one previously reported [35] we couple to three input ports simultaneously using a Pitch Reducing Optical Fibre Array (PROFA) mounted on a fully angle-adjustable stage. The PROFA alignment was optimized to be within 2 dB of the optimal coupling values for all the ports simultaneously. Output coupling is performed with a tapered lensed fibre aligned to one output port at a time. Intrachannel crosstalk penalties The back-to-back reference test case for power penalty measurements is defined by bypassing the chip and emulating insertion loss for the lowest loss port (port 1) with a variable optical attenuator. Intrachannel crosstalk penalties result in a power penalty predicted analytically [33] as PP=−10log 10 (1−2 ) where ε is the ratio of the desired-signal’s power to interfering signals’ powers. Channel decorrelation In order to guarantee correct characterization of the device, the input data channels that originate from a single Pulsed Pattern Generator need to be decorrelated. The data channels coupled to the ports of the device are decorrelated by 0.5-and 1-km-long fibre delays, which ensure that the patterns are relatively shifted between ports by at least 24 kb out of the pattern length of 2 Gb (2 31 −1 PRBS). In the second experiment, the wavelength channels are first decorrelated using the dispersion of a 0.5-km fibre to achieve at least 90-bit relative delay between adjacent wavelength channels. The inputs to the two ports used in this experiment are also decorrelated by a fixed 1-km fibre delay, which guarantees decorrelation between the ports used. How to cite this article: Luo, L.-W. et al. WDM-compatible mode-division multiplexing on a silicon chip. Nat. Commun. 5:3069 doi: 10.1038/ncomms4069 (2014).